Capsule-controlled selectivity of a rhodium hydroformylation catalyst Chemical processes proceed much faster and more selectively in the presence of appropriate catalysts, and as such the field of catalysis is of key importance for the chemical industry, especially in light of sustainable chemistry. Enzymes, the natural catalysts, are generally orders of magnitude more selective than synthetic catalysts and a major difference is that they take advantage of well-defined cavities around the active site to steer the selectivity of a reaction via the second coordination sphere. Here we demonstrate that such a strategy also applies for a rhodium catalyst; when used in the hydroformylation of internal alkenes, the selectivity of the product formed is steered solely by changing the cavity surrounding the metal complex. Detailed studies reveal that the origin of the capsule-controlled selectivity is the capsule reorganization energy, that is, the high energy required to accommodate the hydride migration transition state, which leads to the minor product. Transition metal catalysis is a powerful tool to engender selectivity in chemical transformations, and its importance has been acknowledged by three recent Nobel Prize Awards for homogeneous catalysis. Notably, an increasing number of chemical processes, especially in the fine chemical industry, make use of catalysis as it results in shorter synthetic routes, less waste per quantity of product and overall is economically beneficial [1] , [2] . The properties of a transition metal catalyst are largely determined by the ligands that are coordinated to the metal and, as such, catalyst optimization is traditionally done by modifications to the primary coordination sphere of the metal, that is, by tuning the electronic and steric properties of the ligands that coordinate to the metal centre. To facilitate catalyst design, the properties of ligands have been quantified; for instance, the X-value, the cone angle [3] and bite angle [4] , [5] are nowadays frequently used parameters to describe the electronic properties and the steric bulk of a ligand. Whereas ligand-controlled catalysis has led to a plethora of selective catalysts that can be used for practical synthesis, man-made catalysts do not quite approach the activities and selectivities displayed by enzymes, their natural counterparts. Enzymes are generally two orders of magnitude larger in size, and the mode of operation is quite different. Many of the enzyme-catalyzed reactions that do not involve redox chemistry comprise relatively simple activation of substrates, and high reaction rates are obtained by a combination of effects, including transition state stabilization and protein dynamics [6] . The selectivity of an enzyme is largely controlled by the cavity around the active site which exerts more control over the substrate motions with respect to the active site compared with transition metal complexes that only use the bonding interactions between substrate and active site. As such, the selectivities obtained by enzymatic reactions are generally far beyond those of man-made catalysts. In addition, enzyme performance is modified mostly by changing the environment around the active site rather than the active site itself. As a consequence, tailoring enzymes for synthetic applications also involves modifications of the enzyme cavity, rather than the active site. The catalytic performance of enzymes is nowadays routinely modified by using directed evolution and site-mutagenesis [7] , and also for artificial metallo-enzymes this has been demonstrated to be powerful [8] , [9] . These working principles have also inspired chemists for decades and enzyme mimics have been prepared and studied [10] , [11] , [12] , [13] , [14] to understand them, and also to increase the tool box of methods for performing chemical transformations efficiently. The development in supramolecular chemistry has evolved such that several synthetic systems are now available to also study the reactivity in confined nano-spaces, such as the well-defined cavities of metal-organic frameworks, and (supra)molecular capsules. It has been demonstrated by the pioneering work of Sanders and co-workers [15] , Rebek and co-workers [16] , [17] , [18] , [19] , Fujita and co-workers [20] and Raymond and co-workers [21] that organic reactions that occur in such restricted environments can result in unusual selectivities and rate enhancements. These all are elegant examples in which it has been demonstrated that the activity or selectivity of organic reactions can be controlled by nano-capsules. In this contribution, we show that we can control the regioselectivity of a transition-metal-catalyzed reaction by only changing the shape of the capsule, leaving the actual catalyst identical in all experiments. Importantly, we demonstrate this for the industrially relevant hydroformylation reaction, achieving regio-control in the functionalization of internal alkenes, which is not possible by means of traditional ligand design strategies. The selectivity obtained is qualitatively understood by detailed information on the reaction, obtained via in situ spectroscopy, kinetic analysis and density functional theory (DFT) calculation of the pathways involved, allowing catalysis by rational design of the cavity. Formation of capsules We previously introduced the ligand-template strategy for creating dynamic well-defined cavities around ligand-binding sites and the metal coordinated to such ligands [22] . Upon mixing tris-( meta -pyridyl)-phosphine ((m-py) 3 P) and three equivalents of Zn(II)tetraphenylporphyrin (ZnTPP) in toluene, the assembly forms by selective pyridyl–zinc coordination. The structure is also confirmed in the solid state, as will be clear from data presented in this paper. We considered the application of these types of capsules in the hydroformylation of non-functionalized, linear internal alkenes highly interesting as (1) these challenging substrates are less reactive than the 1-alkenes, (2) they lack functional groups as handles to direct product formation [23] , [24] , [25] and (3) the selective (isomerization-free) functionalization of internal alkenes in general, and to form the aldehyde product in particular, is not yet possible and yet would provide an interesting new route to prepare functionalized alkanes in a selective fashion from available starting materials. Ligand design approaches have so far resulted in catalysts that typically produce a (close to) 1:1 mixture of aldehydes, and generally a considerable amount of isomerized starting material is obtained. The most interesting results up to now are obtained with catalysts based on electron-poor phosphite ligands or rigid bidentate phosphines that effectively catalyze an isomerization–hydroformylation sequence, producing mainly linear aldehydes starting from internal alkenes ( Fig. 1 ) [26] . 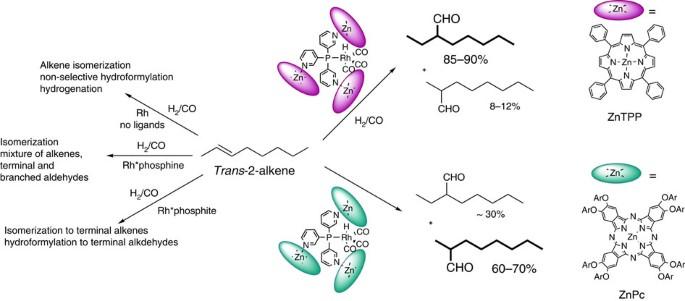Figure 1: Hydroformylation of 2-alkenes. Catalyst obtained by traditional ligand design provide mixtures of products or combine isomerization with hydroformylation. Regio-selective catalysts can be achieved using the encapsulated rhodium catalysts. Figure 1: Hydroformylation of 2-alkenes. Catalyst obtained by traditional ligand design provide mixtures of products or combine isomerization with hydroformylation. Regio-selective catalysts can be achieved using the encapsulated rhodium catalysts. Full size image Kinetic and DFT studies of catalysis In a preliminary study, we found that the rhodium catalyst based on ((m-py) 3 P) as the template-ligand and ZnTPP as the building block displayed remarkable selectivity in the hydroformylation of 2-octene, providing the 3-aldehyde as the major product [27] . In contrast, the non-encapsulated traditional ligand system gave the 1:1 mixture of products. To allow rational design of the nano-environment as a means to control such selectivity we now have carried out detailed studies on the origin of the capsule-induced selectivity. First, we confirmed with in situ high-pressure-infrared spectroscopy [26] that, under the conditions applied, the encapsulated RhH(CO) 3 (m-py) 3 P is the resting state of the reaction indicating a rate determining step early in the cycle (please see Supplementary Note 1 and Supplementary Figs S1, S2 and S3 for the details on the characterization). This was confirmed by the kinetic data that were obtained for this reaction ( Supplementary Fig. S4 and Supplementary Note 2 ), which indeed suggest that the hydride migration from Rh to the coordinated alkene determines the selectivity in this reaction. A DFT study of the catalytic cycle with the encapsulated and the non-encapsulated catalyst analogue was performed, under the consideration of the various catalytic reaction pathways. Starting from the four possible alkene complexes that can form (displayed in Fig. 2a ), there are eight transition states for the hydride migration, finally leading to four pathways for each of the aldehyde products. Taking into account these eight transitions states, the calculations confirm that the selectivity is determined in the hydride migration step. 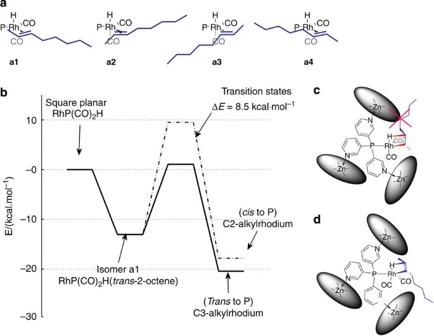Figure 2: Substrate rotation blocked by ZnTPP capsule. The substrate rotation is blocked by the ZnTPP capsule in most of the catalytic pathways leading to 2-aldehyde. (a) The four rhodium-(trans-2-octene) isomer complexes for which the hydroformylation paths were calculated (DFT: Gaussian 03, ONIOM, pbe1pbe/3–21 g** for Zn(porphyrin) complexes (low-level ONIOM) and pbe1pbe/dgdzvp for the rest (high level). (b) The energy diagram of a hydride migration of the isomera1, showing that the pathway towards the 2-aldehyde (dashed line, its scheme shown inc) is much higher in energy than the one leading to the 3-aldehyde (full line, scheme ind) for the ZnTPP-encapsulated catalyst. The schematic drawings of the transition states indicate the important steric interaction of the substrate with capsule. Figure 2b shows that the path to 3-alkylrhodium is much lower in energy than to 2-alkylrhodium, which is the case for three of four Rh-alkene isomers (the complete eight diagrams are shown in Supplementary Fig. S5 ). The product distribution calculated after the hydride migration predicts that the encapsulated catalyst forms preferably the 3-aldehyde product (90%, Supplementary Fig. S6 ), just as was found experimentally (91%). A MATLAB simulation taking into account all DFT-computed reaction constants (based on the energy barriers) and the full catalytic cycle also shows that the 3-aldehyde ( ca. 75%, Supplementary Fig. S6 ) is the main product. These calculations also indicate that detailed understanding of mechanism by which the capsule induces selectivity in this reaction can be found by further analysis of the structural changes of the capsule in the hydride migration step. Figure 2: Substrate rotation blocked by ZnTPP capsule. The substrate rotation is blocked by the ZnTPP capsule in most of the catalytic pathways leading to 2-aldehyde. ( a ) The four rhodium-( trans -2-octene) isomer complexes for which the hydroformylation paths were calculated (DFT: Gaussian 03, ONIOM, pbe1pbe/3–21 g** for Zn(porphyrin) complexes (low-level ONIOM) and pbe1pbe/dgdzvp for the rest (high level). ( b ) The energy diagram of a hydride migration of the isomer a1 , showing that the pathway towards the 2-aldehyde (dashed line, its scheme shown in c ) is much higher in energy than the one leading to the 3-aldehyde (full line, scheme in d ) for the ZnTPP-encapsulated catalyst. The schematic drawings of the transition states indicate the important steric interaction of the substrate with capsule. Full size image In Fig. 3a , we display the X-ray structure of the encapsulated free ligand ((m-py) 3 P) and its DFT-optimized RhHCO 3 L analogue ( Fig. 3b ), from which it is clear that the capsule hardly needs to adjust to accommodate the metal complex, or the hydride migration transition state leading to the 3-alkylrhodium complex and, subsequently, to 3-aldehyde ( Fig. 3c ). In contrast, we found that significant structural changes are necessary to accommodate the transition state of the hydride migration step that leads to the 2-alkylrhodium species (and to the minor 2-aldehyde product), Fig. 3d . As can be seen from the X-ray structure, CH– π interactions between adjacent Zn(TPP) building blocks are present in the parent capsule (the average distance CH– π plane is 2.867 Å, Supplementary Fig. S7 shows the details of these interactions, Supplementary Note 3 relates the previously measured association constants to the cooperativity), and these become weaker or are lost upon capsule distortion. As a consequence, an energy penalty is involved in the capsule reorganization to accommodate the above-mentioned transition state, and therefore the pathway to the 2-aldehyde is blocked. In contrast, the hydride migration transition state that leads to the 3-alkylrhodium (and after completing the cycle, the major 3-aldehyde product) hardly affects the cavity structure, and hence the reaction path to the formation of the observed product is not hindered (for part of the profile, see Fig. 2b , and for the energy required for the capsule reorganization, see Supplementary Fig. S8 ). 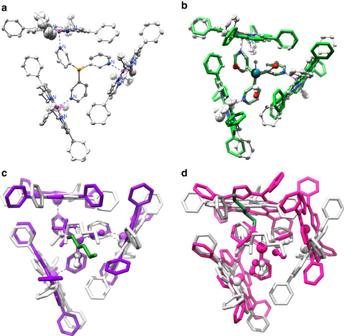Figure 3: Structural analyses. The crystal structure of the tris-(meta-pyridyl)-phosphine·(ZnTPP)3assembly (a) and the overlay with the DFT-calculated structure of the rhodium complex (green inb) showing minimal structural changes. Overlay of the encapsulated catalyst–substrate complexes (white) and the hydride migration transition state to the 3-aldehyde (c, violet; the substrate is green) and the capsule in the TS to the 2-aldehyde (d, magenta, the substrate is green). Figure 3: Structural analyses. The crystal structure of the tris-( meta -pyridyl)-phosphine·(ZnTPP) 3 assembly ( a ) and the overlay with the DFT-calculated structure of the rhodium complex (green in b ) showing minimal structural changes. Overlay of the encapsulated catalyst–substrate complexes (white) and the hydride migration transition state to the 3-aldehyde ( c , violet; the substrate is green) and the capsule in the TS to the 2-aldehyde ( d , magenta, the substrate is green). Full size image Capsule variation This analysis on the basis of the calculations and initial catalysis results suggested to us that modification of the capsule shape could potentially lead to different product distributions. This can easily be achieved by using different Zn(TPP) analogues for encapsulation. Inspection of the X-ray structure would predict that (1) para -, di- meta - or ortho- substitution of the phenyl ring of the porphyrin would disrupt the cavity by steric hindrance, (2) substitution at only one meta -position of the phenyl in principle leaves the shape intact, but may change the CH– π interaction (of the non-substituted meta-H), (3) removing or replacing the phenyl rings with cyclohexyls would also change the interaction. Accordingly, we performed the catalytic reactions using a variety of porphyrin compounds and found most experimental results to be as anticipated (see Fig. 4 and Table 1 ). The distorted capsules provided the product in close to a 1:1 ratio, indicating that most of the cavity effect was lost (entries 8–11). The application of ZnTPP- m,m OMe even displayed a small preference for the production of the 2-aldehyde (entry 8). If ZnTPP- m OMe is applied as the building block to form the encapsulated rhodium catalyst, the result is unaltered in terms of conversion and selectivity in 2-octene hydroformylation as compared with the parent capsule based on ZnTPP (entries 6, 7 and 14, 15). 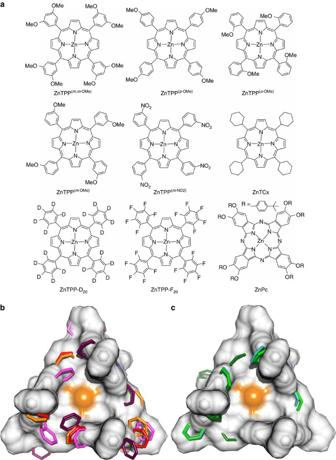Figure 4: Modification of the Zn(porphyrin) building blocks. Modification of the Zn(porphyrin) building blocks affect the capsule structure and the selectivity. (a) Various porphyrin building blocks and their impact on the capsule shape: distortion (b) and minor changes (c). These modifications of the capsule shape have dramatic impact on the selectivity of the encapsulated rhodium catalyst (seeTable 1). Figure 4: Modification of the Zn(porphyrin) building blocks. Modification of the Zn(porphyrin) building blocks affect the capsule structure and the selectivity. ( a ) Various porphyrin building blocks and their impact on the capsule shape: distortion ( b ) and minor changes ( c ). These modifications of the capsule shape have dramatic impact on the selectivity of the encapsulated rhodium catalyst (see Table 1 ). Full size image Table 1 Hydroformylation of alkenes using encapsulated catalysts with various capsule shapes. Full size table In order to evaluate the sensitivity of the system, we also investigated the tetrakis-pentafluorophenyl ZnTPP analogue (ZnTPP–F 20 , entry 12). The capsular catalyst completely loses its selectivity, showing a small preference for the 2-aldehyde product. Moreover, even the smallest changes of the attractive interactions has a visible impact on the selectivity, as was demonstrated by the use of the Zn (tetrakis-(pentadeuterophenyl)-porphyrin) (ZnTPP–D 20 , entry 13). The subtle size differences between the pentaprotophenyl and the pentadeuterophenyl groups, as well as different polarizabilities of the C– 1 H and C– 2 H bonds [28] , [29] , [30] , [31] , [32] , both contribute to the weakening of the CH– π attractions, resulting in the selectivity dropping from 91% (with ZnTPP) to 70% (with ZnTPP–D 20 , entries 6 and 13, respectively). This example highlights the importance of the weak interactions between the porphyrin building blocks of the capsule, contributing to the reorganization energy and hence the selectivity of the enclosed transition metal catalyst. The DFT-optimized structures of the capsules studied using these ZnTPP analogues confirm that the changes in the porphyrin structure indeed had the anticipated impact on the capsule structure. As a measure of the distortion of the cavity, we calculated the average distance of the meta-H position, to the adjacent porphyrin ring, as this is a key interaction in the parent Zn(TPP)-based capsule. As can be seen from the table, this distance correlates well with the selectivity displayed by the catalyst. Minimal deviations of this distance from that observed in the crystal structure are displayed by the ZnTPP- m OMe-based capsule. This is also clearly visible from the overlay plots of the calculated structures (compare Fig. 4b, c ). Interestingly, the capsules with the largest distortion, also gave the largest deviation in terms of selectivity, giving slight preference for the 2-aldehyde. Phtalocyanine-based capsules These results stimulated us to investigate even larger cavities to see if we could push the selectivity even further to the 2-aldehyde product. In order to increase the cavity size significantly, we decided to apply Zn(II)phthalocyanine (ZnPc, Fig. 4a ) as a building block for the capsule formation. These compounds are structurally related to porphyrins, however, without the out-of-plane meso-phenyl groups and with an extended planar surface around the Zn-centre. Detailed characterization, that will be published in a separate paper, show that these building blocks lead to similar 3:1 complexes when mixed with ((m-py) 3 P), and that similar RhH(CO) 3 L resting states could be identified under catalytic conditions, indicating that they react according to a similar pathway. DFT-calculated structures of these ZnPc capsules indicate that the volume of the cavity formed was about five times larger than the parent ZnTPP capsule ( Fig. 5 ). It was anticipated that hydride migration in these capsules could take place in an almost unhindered fashion, so the optimal capsule structure for these systems does not need to adapt to accommodate any of the transition states. Accordingly, the DFT-computed reaction pathways of the hydroformylation of trans -2-octene using the catalyst encapsulated by a simplified ZnPc complex (without the peripheral aryloxy substituents) predicted the 2-aldehyde as the major product. These DFT-predicted results are in an excellent agreement with the experiments, as the ZnPc-encapsulated catalyst led to the formation of 2-aldehyde as major product (60–70%) when 2-alkenes (octene to decene, entries 1–7) were used as substrates. Most importantly, this selectivity is opposite to that displayed by the parent ZnTPP-encapsulated catalyst (87–91% 3-aldehyde for 2-alkenes, entries 6–7), and as the catalyst is the same this shows that the selectivity of the reaction is completely steered by the second shell nano-environment. 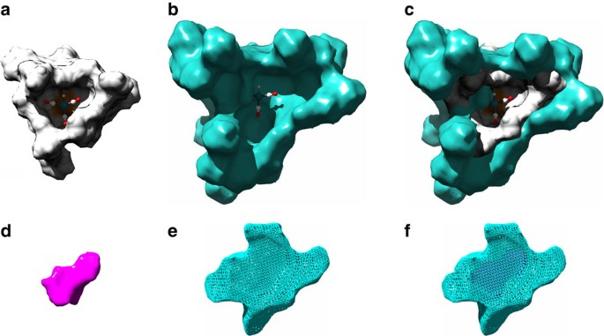Figure 5: Comparison of ZnTPP- and ZnPc-based capsule sizes. (a) ZnTPP-encapsulated catalyst, (b) ZnPc-encapsulated catalyst, (c) overlaidaandb; (d) the cavity insideais much smaller than the one insideb, as can be seen ine. The large cavity of the ZnPc-based capsule most probably allows unhindered motion of the substrate in the capsule, leading to 2-aldehydes as major products, whereas the smaller, ZnTP-based capsule hinders the rotation of the substrate in the paths leading to the 2-aldehyde, resulting in 90% 3-aldehyde as the catalysis product. Figure 5: Comparison of ZnTPP- and ZnPc-based capsule sizes. ( a ) ZnTPP-encapsulated catalyst, ( b ) ZnPc-encapsulated catalyst, ( c ) overlaid a and b ; ( d ) the cavity inside a is much smaller than the one inside b , as can be seen in e . The large cavity of the ZnPc-based capsule most probably allows unhindered motion of the substrate in the capsule, leading to 2-aldehydes as major products, whereas the smaller, ZnTP-based capsule hinders the rotation of the substrate in the paths leading to the 2-aldehyde, resulting in 90% 3-aldehyde as the catalysis product. Full size image The selectivity of transition metal catalysts is traditionally optimized by ligand variation, whereas for the enzymes, the optimization generally relies on modification of the cavity around the active site that should accommodate and orient the substrate prior to its transformation. In this contribution, we show for the first time that such an enzyme-like approach could also apply to transition metal complexes. Throughout the paper, we have used the same catalyst, RhH(CO) 3 (m-py) 3 P, and only changed the nano-environment around it by applying various zinc-based templates for the capsule assembly. Application of these encapsulated rhodium catalysts in hydroformylation of 2-octene shows clearly that the dominant product formed strongly depends on the size of capsule. The application of ZnPc results in a spacious capsule, and the catalyst inside leads to formation of 2-aldehydes as main products (up-to 70%). Encapsulation of the same metal complex using ZnTPP, leading to the smallest capsule of this type so far, results in the formation of 3-aldehyde as the main product (90%). Importantly, our experiments were guided by DFT calculations (in combination with kinetic analysis), which demonstrated that the origin of the selectivity is blockage of the hydride migration pathway to the 2-aldehyde product. Small changes to the porphyrin structure lead to distortion of the capsule, and hence a change in the selectivity in this reaction. Importantly, the selectivity displayed by the encapsulated catalysts is unique, so far there are no traditional catalysts known that can address this selectivity issue. It is anticipated that the strategy outlined in this paper, may be applicable to other unsolved selectivity issues in transition metal catalysis, especially for reactions that involve a selectivity determining migration. In general, we believe that the future generations of transition metal catalysts will increasingly include enzyme-like features in order to achieve selective functionalization of challenging substrate molecules [33] . General Solvents used for pyridyl-phosphine synthesis, catalysis, spectroscopic (HP-FTIR (high-pressure-Fourier transform infrared), ultraviolet–visible) and crystallization experiments were dried and freshly distilled prior to use: toluene and hexane over Na/benzophenone and CH 2 Cl 2 over CaH 2 . Solvents for synthesis and column chromatography of porphyrins were used as obtained from the supplier. The deuterated solvents were dried and degassed using the freeze–pump–thaw technique and kept under Ar over 4 Å molecular sieves. 1-Octene and trans -2-octene were purified by filtration over a plug of alumina and degassed by bubbling Ar. All handling and manipulations, except synthesis and chromatographic purification of porphyrins, were performed under oxygen- and water-free atmosphere (dinitrogen, Ar or synthesis gas). Infrared spectra were recorded on the Nicolet Nexus 670 FT-IR spectrometer operated by Omnic 6.2 Software; ultraviolet–visible measurements were performed on the Hewlett-Packard 8453 and the Varian Cary 4 spectrophotometer. Gas chromatography (GC) analysis were performed on the Shimadzu GC-17A chromatograph equipped with an flame ionization detector using a 30 mm long column with 0.32 mm diameter and dimethylsiloxane cross-linked phase of 3 μm thickness. Syntheses The porphyrins were synthesized according to the published procedures, in general following the Rothemund–Adler–Longo methodology [34] , and the metallation of the free-base porphyrins was performed by refluxing the porphyrins with zinc acetate in a 5:1 methanol/chloroform mixture. Tris-( meta -pyridyl)-phosphine ligand was prepared using the previously published procedure [35] . ZnII(phthalocyanine) ZnPc was synthesized from the 4,5-bis-(4-t-butylphenoxy)-phthalonitrile and zinc(II)-acetate catalyzed by DBU (1,8-diazabicyclo[5.4.0]undec-7-ene) by heating in 1-pentanol, according to the published procedures [36] . The NMR data of all synthesized compounds were in agreement with already published characterization data and will therefore not be repeated here. Crystallization The crystallization of the supramolecular capsule assembly P( m -pyridyl) 3 *3ZnTPP was achieved by a slow (7–14 days) hexane diffusion into a saturated toluene solution of ZnTPP and the phosphine in the 3:1 ratio. ZnTPP (62 mg, 92 μmol) and tris-( meta -pyridyl)-phosphine (8.09 mg, 30.5 μmol) were dissolved in as little toluene (5.0 ml) as possible under heating (up to 100 °C) and in the ultrasonic bath. The hot, saturated solution was filtered via an HPLC syringe filter into a scratched Schlenk tube ( ca. 1.5 ml) and was top-layered with cold hexanes ( ca. 2.0 ml). The tube was protected from light by Al-foil and was left at ambient temperature (20–25 °C). C 147 H 96 N 15 PZn 3 +disordered solvent, Fw=2299.47 (Derived values do not contain the contribution of the disordered solvent. ), red needle, 0.48 × 0.20 × 04 mm 3 , monoclinic, C2/c (no. 15), a =53.9189(8), b =29.3288(2), c =18.7501(3) Å, β=96.069(2)°, V =29484.8(6) Å 3 , Z =8, D x =1.04 g cm −3 (Derived values do not contain the contribution of the disordered solvent. ), μ=0.54 mm −1 (Derived values do not contain the contribution of the disordered solvent.). In total, 139,949 reflections were measured on a Nonius KappaCCD diffractometer with rotating anode and graphite monochromator ( λ =0.71073 Å) up to a resolution of (sin θ / λ ) max =0.61 Å −1 at a temperature of 150(2) K. Intensity data were integrated with the Eval14 software [37] . Absorption correction and scaling was performed based on multiple measured reflections with SADABS [38] (0.50–0.75 correction range). In total, 27,415 reflections were unique ( R int =0.141), of which 13,724 were observed [ I >2 σ ( I )]. The structure was solved with direct methods using the program SHELXS-97 (ref. 39 ) and refined with SHELXL-97 against F 2 of all reflections. The structure contains voids (9,604.4 Å 3 per unit cell) filled with disordered solvent molecules. Their contribution to the structure factors was secured by back-Fourier transformation using the SQUEEZE routine of the PLATON package [40] , resulting in 2,750 electrons per unit cell. One thousand four hundred and ninty-five parameters were included in the least-squares refinement. Non-hydrogen atoms were refined with anisotropic displacement parameters. Hydrogen atoms were introduced in calculated positions and refined with a riding model. Seventy-five restraints were used for the refinement of the ill-defined phenyl ring C333–C383 (restraints for isotropic behaviour and for the flatness of the ring). R1/wR2 [ I >2 σ ( I )]: 0.0594/0.1410. R1/wR2 [all refl. ]: 0.1248/0.1578. S =0.908. Residual electron density between −0.56 and 0.70 e Å −3 . Geometry calculations and checking for higher symmetry was performed with the PLATON program [40] . HP-FTIR spectroscopy HP-FTIR spectroscopy experiments were conducted using an autoclave adapted for infrared measurements of the reaction mixture [41] , which was cleaned, dried, tested for leaks (pressurized with 40 bar hydrogen for 16 h), and flushed (3 × 15 bar) with syngas prior to every use. These experiments were performed under conditions identical to those under which the catalytic experiments were done, with the only exceptions being the solvent and substrate concentration: dichloromethane was used instead of toluene and 200 equivalents substrate ( trans -2-octene) instead of 500. For details on the results please refer to Supplementary Note 1 . Kinetics studies The kinetics of the trans -2-octene hydroformylation by the ZnTPP-encapsulated rhodium catalyst were studied at 40 °C by measuring the gas uptake at various pressures and three syngas compositions using the AMTEC robot during the reaction. The concentrations of the catalyst and substrate were identical to those used in the catalysis experiments; however, the reaction volume was 8.0 instead of 4.0 ml, so that the amounts of compounds used for a single run were double of those used in the normal catalysis runs. ZnTPP, phosphine and diisopropylethylamine (DIPEA) were stirred in toluene (under Ar) for 30 min at room temperature, before Rh(acac)(CO) 2 and trans -2-octene were added. Portions of 8.0 ml of this stock solution were transferred into the stainless steel autoclaves (all under Ar), which were flushed with syngas (3 × 15 bar) and pressurized to 20 bar. Gas-uptake measurement started upon finished pressurization of all autoclaves. Three syngas compositions were employed, at four different total pressures: (1) CO/H 2 =1:1, P =10, 20, 30 and 40 bar; total reaction time 90 h; (2) CO/H 2 =1:2, P =15, 23, 30 and 45 bar; total reaction time 50 h; (3) CO/H 2 =2:1, P =8, 15, 23 and 30 bar; total reaction time 45 h. In addition, a series of four experiments at CO/H 2 =1:1 (at 10, 20, 30 and 40 bar) was performed with 0.60 mol l −1 substrate (in other experiments it was 0.25 mol l −1 ). Upon de-pressurization, n -tributylphosphite was added for quenching, and the samples were analysed by GC in a usual way (reaction mixture diluted with methylene chloride without product isolation). The results are shown in Supplementary Table S1 and in Supplementary Fig. S9 . The raw data, in ml gas, was correlated with conversion using the final values of either, so that the data pairs (substrate) concentration versus time could be reconstructed. These data vectors were subject to as little numeric manipulation as possible; the data points were smoothed, in order to perform numerical differentiation and obtain the substrate consumption rates ( r=− (d c/ d t )). Using the reaction progress kinetics analysis approach [42] , we were able to determine the reaction rate orders in reactant concentrations. The raw gas uptake data were not fitted to analytical expressions describing potential rate laws. Instead, the data were numerically differentiated to obtain the reaction rate (at any moment), and the rate orders in CO ( m ) and H 2 ( n ) were obtained by fitting the rate versus partial pressure to the corresponding equations: r = K * p m (CO) (for p (H 2 )=const.) and r = K * p n (H 2 ) (for p (CO)=const.). Broken rate orders were found in all three reactants: −0.9 in CO, +0.7 in H 2 and +0.8 in trans -2-octene. In addition, plot of the graphical rate equation was done in order to investigate potential decomposition or deactivation phenomena during catalysis ( Supplementary Fig. S10 ). Geometry optimizations The geometry optimizations were performed using Gaussian 03 Rev. C.02 (ref. 43 ) on the Dutch national computing cluster Lisa, which was installed by SARA, The Dutch National High Performance Computing and e-Science Support Center SARA ( http://www.sara.nl/aboutsara/aboutsara_pr_eng.html ). The equilibrium geometry optimizations of the non-encapsulated structures were performed using the hybrid functional of Perdew et al . [44] (pbe1pbe) with DGauss double zeta double valence polarization [45] (dgdzvp) all-electron basis set. The computations were followed by an additional frequency calculation after the optimization, in order to obtain the free energy of the system (per default it was computed at 298 K). The transition states were found by performing the relaxed potential energy scan computation along the reaction coordinate (backwards for the hydride migration and oxidative addition of hydrogen, forwards for the alkyl (CO) migratory insertion and reductive elimination of the aldehydes) in order to locate the preliminary, near-saddle point structure. Next, the transition state search with calculation of forces at every search step led to the saddle point structure in 3–5 steps. All transition state structures displayed an imaginary frequency in their infrared spectra, describing the motion of the bond breaking and/or the bond forming event in the transition state. The free-energy diagrams displayed in Supplementary Table S2 and Supplementary Fig. S11 were obtained by summation of the free energies (at 298 K) of the molecules participating in one catalytic cycle: the rhodium catalyst, CO, H 2 , substrate and/or products. Two-layer ONIOM [46] method was used to compute large structures, with the hybrid functional pbe1pbe with the DGauss double zeta double valence polarization [45] (dgdzvp) all-electron basis set for high-level layer, and with 3–21 g** as basis set for low-level layer in ONIOM. The cut between the layers was between the N atom of the pyridyl moieties of the phosphine and Zn of the Zn(tetraphenylporphyrin) complexes, no dummy atoms were used. The optimized non-encapsulated structures of the model catalyst were used to construct the ZnTPP-encapsulated catalyst molecules by simply replacing the calculated phosphine molecule with the crystal structure of the supramolecular capsule. The energies of the transition states were computed by performing a normal geometry optimization of the structure in which the atoms participating in the transition state were kept frozen (structure from the previously calculated non-encapsulated complex), whereas all the other atoms and the capsule were allowed unrestricted movement. The self-consistent field (SCF) energies obtained in calculations were corrected for entropy contributions to energy (at 298 K) in the reaction steps consuming, or creating a molecule by +10 and −10 kcal mol −1 , respectively. The energies obtained in this way and the corresponding diagrams are shown in Supplementary Fig. S5 and Supplementary Table S3 . The energies of the capsule during the catalytic cycle were obtained by calculating the single-point energies of the previously optimized structures, from which all atoms except those belonging to the supramolecular capsule P( m -pyridyl) 3 *3ZnTPP were removed. The results are presented in Supplementary Table S4 . All the calculated structures are available online as .xyz files (see Supplementary Data 2 ). The construction of the kinetics simulation was done in MATLAB (R2010a, The Mathworks Inc.), SIMBIOLOGY module, using the DFT-calculated data. The constants of all the forward and backward reactions in the catalytic cycle were calculated using the activation energies obtained from DFT and the Arrhenius’ equation. These microconstants were fed into the kinetics model, which used the simple mass action law to describe the reaction rates. The concentrations of rhodium catalyst and the substrate in the model were identical to those used in experiments, 0.5 mmol l −1 and 0.25 mol l −1 , respectively. The concentrations of CO and hydrogen were set at a constant value of 0.10 mol l −1 (ref. 47 ). The results of the simulation of the non-encapsulated and the encapsulated catalyst, both of the full catalysis cycle and right after the hydride migration step are displayed in Supplementary Fig. S6 . Molecular graphics images were produced using the UCSF Chimera package from the Resource for Biocomputing, Visualization and Informatics at the University of California, San Francisco [48] . The online utility Voss Volume Voxelator ( http://3vee.molmovdb.org/ ) was used to calculate the volume of the capsule (with 2 Å probe radius) and of the cavity (with 12 Å large and 1.2 Å small probe radius) wherein the catalyst is situated [49] . Catalytic evaluation Catalytic experiments were performed in mini-4-autoclaves connected to the same high-pressure line, allowing four reactions to be ran in parallel under the same pressure. Before each run the autoclaves were evacuated, flushed with nitrogen and tested for leaks at 35 bar syngas or hydrogen. Typically, Zn(II)porphyrin complexes were weighed directly in the glass inserts (with a magnetic stirring bar) of the autoclaves, which were then closed, set under inert atmosphere and filled with stock solutions (in toluene, DIPEA neat) of the ligand, DIPEA, Rh(acac)(CO) 2 , the substrate and was topped with toluene to 4.0 ml total volume. Alternatively, stock solutions of Zn(II) complexes were used instead of weighing them directly. The closed autoclaves were flushed with syngas (3 × 25 bar), pressurized to 20 bar (CO/H 2 =1:1), immersed into an oil bath tempered at 25 °C and stirred. After the desired reaction time was reached, the pressure was released, the reactor flushed with dinitrogen, opened and the reaction quenched with a few drops of n -tributylphosphite. The reaction mixture (50 μl) was diluted with dichloromethane and injected into the GC directly without work-up or product isolation. Typical amounts of reactants used are given in Supplementary Table S5 . Accession codes: The X-ray crystallographic coordinates for structures reported in this Article have been deposited at the Cambridge Crystallographic Data Centre (CCDC), under deposition number CCDC 852581. These data are provided in Supplementary Data 1 or can be obtained free of charge from The Cambridge Crystallographic Data Centre via www.ccdc.cam.ac.uk/data_request/cif . How to cite this article: Bocokić, V. et al . Capsule-controlled selectivity of a rhodium hydroformylation catalyst. Nat. Commun. 4:2670 doi: 10.1038/ncomms3670 (2013).